Emerging land use practices rapidly increase soil organic matter The loss of organic matter from agricultural lands constrains our ability to sustainably feed a growing population and mitigate the impacts of climate change. Addressing these challenges requires land use activities that accumulate soil carbon (C) while contributing to food production. In a region of extensive soil degradation in the southeastern United States, we evaluated soil C accumulation for 3 years across a 7-year chronosequence of three farms converted to management-intensive grazing. Here we show that these farms accumulated C at 8.0 Mg ha −1 yr −1 , increasing cation exchange and water holding capacity by 95% and 34%, respectively. Thus, within a decade of management-intensive grazing practices soil C levels returned to those of native forest soils, and likely decreased fertilizer and irrigation demands. Emerging land uses, such as management-intensive grazing, may offer a rare win–win strategy combining profitable food production with rapid improvement of soil quality and short-term climate mitigation through soil C-accumulation. Soils represent the largest terrestrial C reservoir, containing 2,300 Pg of soil organic carbon (SOC) down to 3 m (ref. 1 ). Agricultural cultivation has likely decreased soil C stocks by one-half to two-thirds, with a cumulative loss near 30–40 Mg C ha −1 (ref. 2 ) that has likely contributed 78±12 Pg of C to the atmosphere as carbon dioxide (CO 2 ) [3] . Lower SOC abundance also has a direct impact on soil productivity. Soil organic matter (SOM) enhances soil nutrient-retention, water-holding capacity (WHC) and facilitates healthy microbial communities essential for sustaining high levels of food production [4] . Land-management strategies that sequester C and improve soil quality can potentially reverse soil degradation [5] ; if they can also sustain food production then they deserve careful consideration. The accumulation of C through land management has the potential to offset up to one-third the annual increase in atmospheric CO 2 (ref. 3 ). The most rapid C accumulation is achieved in (sub)tropical aggrading forests or plantations, which have aboveground C accumulation rates as high as 30 Mg ha −1 yr −1 (ref. 6 ) that can be sustained through wood harvest and conversion to building materials. The highest rates of belowground C accumulation occur when land is converted to grassland ecosystems [7] , [8] , [9] , [10] , [11] . Grasses allocate substantial C belowground and can extend their root structures to great depths, leading to thick soil horizons rich in organic matter. Many studies have quantified SOM increases following conversion to grasslands, native prairies and through implementation of conservation tillage, cover crops or perennialization of agroecosystems [3] . Accumulating C in the soil has additional benefits of higher nutrient retention and water-use efficiency—hence improving the sustainability of soil-based agriculture and forestry. Converting tilled cropland to grazed pasture can drive substantial SOC accumulation [12] , [13] while providing food and economic return for a landowner. Intensive grazing systems, such as those studied here, have been tested and used extensively in temperate regions of Australia and New Zealand, and the increases in soil C content and benefits of higher soil nutrient status are well documented [14] , [15] , [16] , [17] . Optimizing either pasture fertilization, irrigation or grazing intensity can each improve C accumulation rates by up to 0.5 Mg C ha yr −1 (ref. 9 ). Intensive pasture management has yielded rates of C accumulation as high as 2.9 Mg C ha −1 yr −1 following the conversion from cropland [13] ; the intensive management required is most economical for high-value end products, such as milk and dairy products. The potential SOM and CO 2 -sequestration benefits of investing in pasture-based land management are likely greatest in highly degraded soils in warm subtropical climates that facilitate long pasture-growing seasons. Highly weathered soils of the subtropics are particularly sensitive to SOM amounts since they often lack minerals, such as 2:1 layer aluminosilicates, with high-nutrient-retention capacity [18] . A century of intensive tillage techniques has exacerbated SOM loss and soil erosion on the highly weathered subtropical soils in the southeastern United States [19] , [20] . However, the long-growing seasons, relatively inexpensive land, regional milk supply shortfalls and high return on investment have fuelled an expanding dairying farming boom [21] , [22] with ∼ 4,000 ha of row crop converted to management-intensive grazing farms in Georgia alone since 2005 (co-author Hancock, personal communication). We sought to determine how fast and how much soil C accumulates following conversion of row crop agriculture to management-intensive grazed pastures in the southeastern United States. We quantified the magnitude and direction of SOC stocks by sampling across grazed pastures established in 2006, 2008 and 2009, defining a chronosequence of land-use change. These pastures were established on land farmed for cotton and peanuts using conventional tillage techniques for the last 50 years, resulting in a SOC content of ∼ 0.5% in the surface horizons ( Supplementary Fig. 1 ). We sampled soil pits and replicated soil cores over 2 years across all pastures and measured soil C, δ 13 C, and soil bulk density. Rapid soil C accumulation Here we report a rapid rate of soil C accumulation accompanying conversion of row crop agriculture land to intensively grazed pastures ( Fig. 1 ) that is on par with the global record for soil C accumulation rate associated with tropical grasslands in Brazil [23] . Fisher, et al. [23] illustrated that the introduction of deep-rooting African grasses to lowland savannas in tropical South America drives C accumulation rates of 7.1 Mg C ha −1 yr −1 and suggested that other fields may have rates as high as ∼ 13 Mg C ha −1 yr −1 (refs 23 , 24 , 25 ). In our pastures, we find that peak C accumulation occurs 2–6 years after pasture establishment with a gain of 8.0±0.85 Mg C ha −1 yr −1 ( r 2 =0.88, P <0.0001) in the upper 30 cm of soil ( Fig. 2 ). Following an apparent lag in the first 2 years, the most recently established farm (converted in 2009) accumulated C at 4.6 Mg C ha −1 yr −1 ( r 2 =0.79, P =0.0184), the middle-established farm (converted in 2008) accumulated C at an average rate of 9.0 Mg C ha −1 yr −1 ( r 2 =0.80, P =0.0395), while the earliest-established farm (converted in 2006) accumulated C at 2.9 Mg C ha −1 yr −1 ( r 2 =0.97, P =0.1125) before an apparent decline in the accumulation rate at 6.5 years following conversion. In all cases, detectable increases in C accumulation were limited to the upper 30 cm ( Supplementary Figs 1 and 2 ), with variability below 30 cm yielding an integrated C accumulation rate of 7.1±2.7 Mg C ha −1 yr −1 in the top metre ( Supplementary Fig. 3 ). This suggests that accumulation at depth may require a longer timeframe or a shift in management practices. 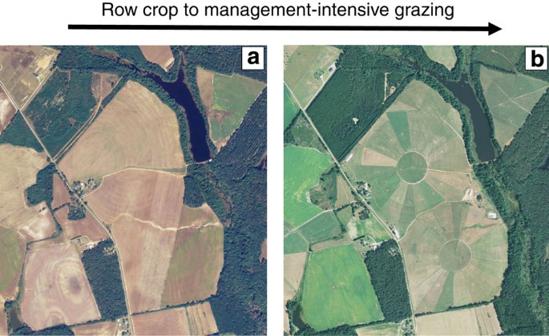Figure 1: Land use shift from row crop to management-intensive grazing. Aerial photographs of the Wrens Farm (Site ID: 2006) taken in 2006 (a) before conversion to management-intensive grazing system and (b) in 2013,∼7 years after land conversion. Figure 1: Land use shift from row crop to management-intensive grazing. Aerial photographs of the Wrens Farm (Site ID: 2006) taken in 2006 ( a ) before conversion to management-intensive grazing system and ( b ) in 2013, ∼ 7 years after land conversion. 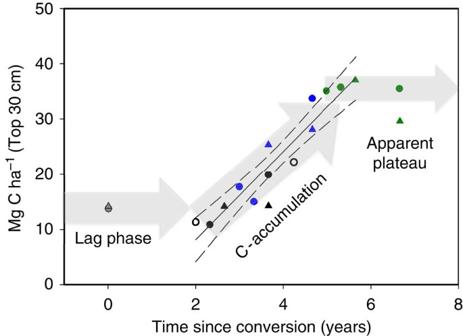Figure 2: Soil carbon rapidly increases with conversion of row crop to intensive grazing. Soil carbon (Mg C ha−1) content shown for the top 30 cm of farms converted in 2006 (green symbols), 2008 (blue symbols) and 2009 (black symbols) and a control farm currently in row crop (grey symbols). Samples from soil pits and soil cores are distinguished by circles and triangles, respectively; open versus closed black circles are from different locations on the 2009 farm. The linear regression (solid line:r2=0.88,P<0.0001) and 95% confidence intervals (dashed lines) are for data between 2 and 6 years since conversion only. The grey-shaded arrows represent our interpretation of soil carbon change in this system on the basis of current data. Full size image Figure 2: Soil carbon rapidly increases with conversion of row crop to intensive grazing. Soil carbon (Mg C ha −1 ) content shown for the top 30 cm of farms converted in 2006 (green symbols), 2008 (blue symbols) and 2009 (black symbols) and a control farm currently in row crop (grey symbols). Samples from soil pits and soil cores are distinguished by circles and triangles, respectively; open versus closed black circles are from different locations on the 2009 farm. The linear regression (solid line: r 2 =0.88, P <0.0001) and 95% confidence intervals (dashed lines) are for data between 2 and 6 years since conversion only. The grey-shaded arrows represent our interpretation of soil carbon change in this system on the basis of current data. Full size image Why we observe high rates of soil C accumulation Soil δ 13 C values are an efficient tracer of this land-use change. The 50+ years of C3 cotton and peanut cultivation established soil δ 13 C values much lower than the major C inputs from grazed pasture grasses, including manure ( δ 13 C=−14.88) and roots ( δ 13 C=−20.03) from the C4 bermudagrass that comprises the bulk of warm season forage on these farms ( Supplementary Fig. 4 ). Consistent with this, the farm exhibiting the highest C accumulation rate also exhibited large changes in δ 13 C, while the farm established in 2006 showed little to no change in δ 13 C over the 2-year study period. However, the farm established in 2006 had root mass abundance (standing stocks) two to three orders of magnitude higher than the more recently established farms ( Supplementary Table 1 ), suggesting high belowground C cycling from root turnover. The transition from crop to pasture systems results in an average 19% increase in soil C stocks [26] . In our intensively grazed systems, we report an ∼ 75% increase in C stocks within 6 years of conversion. This high C accumulation rate stems from year round intensive forage/grazing management techniques on sandy soils with an initially low soil C content due to past conventional-till row crop agriculture. The pastures in this study are managed for maximum forage production; employing N fertilization, irrigation and selective rotational grazing designed to optimize forage digestibility and protein content. These forage-management techniques are precisely those suggested to increase SOM in pasture systems [13] and when they are applied to soils with degraded SOC content, such as soils in the southeastern United States, rapid C accumulation ensues. Consequences for soil quality In addition, the establishment of intensively grazed pastures improved soil quality by increasing soil cation exchange capacity (CEC) and WHC during the 5 year of transition documented by our chronosequence ( Fig. 3 , Supplementary Figs 5 and 6 and Supplementary Table 2 ). CEC increased by 95% in the top 30 cm for an average rate of 44 meq g −1 yr −1 , while WHC increased by 34%. These soil improvements should reduce the need for fertilizer and water inputs and may also mitigate nitrogen (N) losses from the agricultural system. In a companion study on the oldest chronosequence farm, only half of the 620 kg ha −1 of N inputs (silage, hay, grain and mineral fertilizer) were accounted for as N outputs (milk, N 2 O, NH 3 and leached NO 3 ) with the balance presumably sequestered in the SOM pool or lost via denitrification [27] . 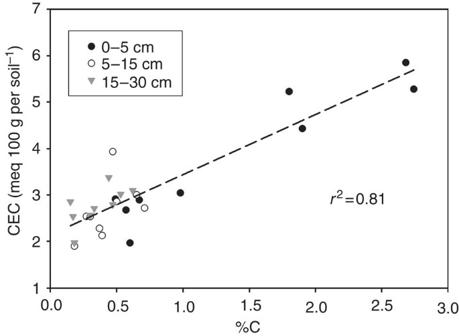Figure 3: The relationship between percent soil C and cation exchange capacity. The relationship is shown at different soil depths along the chronosequence. Soil CEC increases with soil C accumulation. The dashed line is a linear regression of the data (P<0.001). Figure 3: The relationship between percent soil C and cation exchange capacity. The relationship is shown at different soil depths along the chronosequence. Soil CEC increases with soil C accumulation. The dashed line is a linear regression of the data ( P <0.001). Full size image Six years after conversion, our data suggest that an apparent plateau in SOC accumulation occurs at ca. 38 Mg C ha −1 in the top 30 cm, which is consistent with peak SOC stocks in the region [13] , [20] , [28] . C stocks as high as 51 Mg C ha −1 (top 20 cm) have been measured in a bottomland Piedmont forest soil (ref. 20 and references within), suggesting that C may continue to accumulate in these intensively grazed pastures over the millennial scales at slower rates [29] . In New Zealand pastures, soil C stocks have been estimated as high as 109 and 138 Mg C ha −1 (refs 14 , 17 ), and once these soils reach a higher SOC level they can become susceptible to C loss if management changes [15] . Total C stock will be determined by grass productivity, soil physical and biological attributes, and the degree of physical disturbance, which can all change with future management [11] , [20] , [25] . Extrapolation of results The C-accumulation benefits of adopting management-intensive grazing practices are notable. We estimate that if just 10% of the 9 million hectares [30] of cropland in the southeastern United States (average C stock: 10 Mg C ha −1 ) were converted to management-intensive grazing land, ∼ 4.5 Tg of C would be accumulated per year. Assuming peak SOC stocks in the top 30 cm were reached at 40 Mg C ha −1 , this accumulation would continue for a minimum of 6 years, reaching a regional accumulation of 27 Tg C. On the basis of a whole farm C-cycle analysis, C accumulation appears to offset methane emissions [31] during the rapid soil C accumulation phase yielding net C-sequestration rates of ∼ 1.6 Mg C-CO 2 equivalents ha −1 yr −1 or ∼ 5,805 kg CO 2 equivalents ha −1 yr −1 (see Methods section for calculation details). As the C accumulation rate declines these farms will become net C-emitting—similar to all dairy production—because of ruminant methane emissions. However, the substantial soil-quality benefits of higher organic matter remain and will likely increase the sustainability of dairy production using management-intensive grazing. The expansion of this emerging land use practice on previously tilled, row crop land may improve soil quality regionally and could mitigate climate change via rapid increases in soil C. Two daunting challenges facing humanity are feeding a growing population and curtailing the impacts of climate change [5] . Alternative land use activities that reduce environmental degradation (for example, erosion, excess fertilizer and water demand) as well as provide economically viable food can provide a win–win scenario. There are considerable economic incentives for converting irrigated row crop land to grazed pastures used for dairy [22] , especially in warm climates where rainfall is sufficiently high. This practice could vastly improve soil quality [4] and serve as a C sink; however, the magnitude of SOC changes will depend on farm inputs (fertilizer, irrigation and pasture species), pasture management techniques [32] and specific soil conditions. Our results demonstrate that pasture-based intensively grazed dairy systems may provide a near-term solution for agricultural lands that have experienced soil-C loss from previous management practices. Emerging land uses, such as management-intensive grazing, offer profitable and sustainable solutions to our needs for pairing food production with soil restoration and C sequestration. Site description The three farms used in this study were within 40 km of each other on the eastern coastal plain in Burke and Jefferson Counties, Georgia, USA. Soils in this region are deep, well-drained, fine or fine-loamy Kandiudults formed on Coastal Plain sediments and are common to the geographic region. The average annual temperature in this region is 17 °C and annual precipitation is 1,224 mm yr −1 (University of GA Environmental Monitoring Network, 1915–2003). From April to November, evapotranspiration exceeds rainfall and farms irrigate with high-quality aquifer water to meet pasture needs. Forage species in the pasture systems include a hybrid of bermudagrass and stargrass ( Cynodon dactylon (L.) Pers. × C. nlemfuensis Vanderyst; cv. ‘Tifton 85’) as a perennial forage base (grown May through October) that is over-seeded in the fall with annual ryegrass ( Lolium multiflorum Lam. ; cv. ‘Big Boss’, ‘Marshall’ and/or ‘Feast’). Individual paddocks received stock densities ranging from 75 to 150 animal units per hectare during any given 12-h period. Dairy cattle were rotated among 45–60 paddocks (depending on farm layout) twice daily, completing a cycle of grazing all paddocks within 15–45 days, depending on time of year, growth rate and quality of the forage, and the nutritional needs of the herd. Soil characteristics and sampling procedures Soils are classified in the Orangeburg (Fine-loamy, kaolinitic, thermic Typic Kandiudults), Dothan (Fine-loamy, kaolinitic, thermic Plinthic Kandiudults) or Faceville (Fine, kaolinitic, thermic Typic Kandiudults) series and the dominant soil minerals are kaolinite, hematite and quartz. Soils were sampled in April, August and December 2011 and December 2012 by genetic horizon from 1 m pits for soil analyses and bulk density ( Supplementary Tables 2–4 ). Soils were sampled from the bottom of the pit to the top to reduce contaminating subsurface horizons with surface litter. Stainless steel cores were pushed horizontally into pit horizons, removed and dried at 105 °C to determine bulk density. CEC and WHC were determined on pit sample horizons within the top 30 cm. To assess spatial variability, replicate soil cores (five cores composited and replicated six times) were sampled (0–30 cm) at each site on December 2011 and December 2012 ( Supplementary Fig. 7 , Supplementary Table 5 ). A row crop (for example, cotton, corn and peanut rotations) farm on similar soil to grazing dairies was sampled to approximate pre-conversion soils. The row crop farm used in this study was adjacent to the middle-aged (2008) farm and representative of row crop practices in the region. Soil analyses Soils were sieved (2 mm) and fine roots and plant material that passed through the sieve were handpicked and static electricity was used to remove abundant fine roots in the 0–5 cm horizon. Soil C and δ 13 C was assessed by finely grinding samples with a zirconium mortar and pestle and analysed with a coupled continuous-flow elemental analyser—isotope ratio mass spectrometer (Carlo-Erba 1108 EA interfaced to a Thermo-Finnigan Delta Plus XP IRMS). Percent carbon was calculated to an areal basis using bulk density measurements. Bulk density was determined on soils collected in August 2011, December 2012 and July 2013 (youngest farm only) using open-core steel rings (7.5 cm depth × 7.5 cm diameter). For the April 2011 sampling, bulk density was collected using 3.4 cm depth × 8.5 cm diameter cores with one end sealed, which gave abnormally high values in some horizons. Because of this, for the middle-aged farm and the youngest farm, we used the August 2011 bulk density values in our April 2011 calculations ( Supplementary Table 3 ). A homogenized soil sample (air-dried and 2-mm sieved) was sent to the University of Georgia Soil, Plant, and Water Laboratory for chemical analysis. For each sample, P, K, Ca, Mg, Mn, Fe and Zn were extracted using the Mehlich I procedure [33] , [34] , [35] and simultaneously determined using an Inductively Coupled Plasma (Thermo Jarrell-Ash Enviro I ICAP, Fraklin, MA). Soil pH was measured in a 1:1 soil:CaCl 2 (0.01 M) suspension. Particle size analysis was performed using the rapid hexametaphosphate method [36] . Briefly, 3% hexametaphosphate was added to air-dried soils (2-mm sieved) and used as a dispersal agent, followed by fractionation and quantification of each particle size by sieving. CEC was measured using a modified, unbuffered salt extraction method [37] , and exchanged NH 4 + was analysed colorimetrically (Alpkem RFA-303) [38] . WHC was measured by applying the appropriate pressure for field capacity (0.1 bar) and wilting point (15 bar) for sandy soil textures [39] . Belowground root standing stock estimates Coarse roots were defined as those that were greater than 2 mm and fine roots were less than 2 mm. All coarse roots were handpicked from >2 mm sample, washed in DI water, lyophilized and quantified by mass. This value was then divided by the total mass of soil it was sieved from and reported on a per 100-g soil basis. Fine roots were handpicked from a 100-g subsample for no more than 45 min, with static electricity and flotation on DI water used to remove abundant fine roots in the 0- to 5-cm horizons at the termination of the time period. All samples were then washed, lyophilized and massed. Values of coarse and fine roots were combined to give a total root mass per 100-g soil sample. Whole farm C sequestration calculation Belflower et al. [31] compared the whole-farm C-cycle balance between a Georgia conventional dairy farm and one of the intensively grazed dairies used in our study (Farm Site ID-2008 reported here) using the Integrated Farm System Model. They reported an emission rate of ∼ 2,350,700 kg CO 2 equivalents per year for this farm. By factoring in our estimates of soil C accumulation (8.0 Mg C ha −1 yr −1 ), we calculate a net soil sequestration rate of ∼ 1.58 Mg C-CO 2 equivalents ha −1 yr −1 or ∼ 5,805 kg CO 2 equivalents ha −1 yr −1 . Further, we estimate that a soil C accumulation rate of 6.4 Mg C ha −1 yr −1 or higher is required for these systems to serve as a net C sink. While such a high rate cannot be maintained indefinitely following conversion, intensively grazed pasture does meet this criterion for at least an initial 5-year period following land use change. Statistics Linear regression models were performed in JMP 10.0 (SAS Institute, Cary, NC). An alpha level of 0.05 was used to determine significant effects. How to cite this article: Machmuller, B. M. et al. Emerging land use practices rapidly increase soil organic matter. Nat. Commun. 6:6995 doi: 10.1038/ncomms7995 (2015).